Action-value comparisons in the dorsolateral prefrontal cortex control choice between goal-directed actions It is generally assumed that choice between different actions reflects the difference between their action values yet little direct evidence confirming this assumption has been reported. Here we assess whether the brain calculates the absolute difference between action values or their relative advantage, that is, the probability that one action is better than the other alternatives. We use a two-armed bandit task during functional magnetic resonance imaging and modelled responses to determine both the size of the difference between action values ( D ) and the probability that one action value is better ( P ). The results show haemodynamic signals corresponding to P in right dorsolateral prefrontal cortex (dlPFC) together with evidence that these signals modulate motor cortex activity in an action-specific manner. We find no significant activity related to D . These findings demonstrate that a distinct neuronal population mediates action-value comparisons, and reveals how these comparisons are implemented to mediate value-based decision-making. For behaviour to remain adaptive a decision-maker must be able to rapidly establish the best action from multiple possible actions. Such ‘multi-armed bandit’ problems are, however, notoriously resistant to analysis and typically hard to solve when employing realistic reward distributions [1] , [2] , [3] . Understanding the variables we compare to make choices and how we select the best option has, therefore, become an important goal for research into adaptive systems in economics, psychology and neuroscience [4] , [5] , [6] , [7] , [8] . It is important to note that choosing between different actions often occurs in the absence of cues predicting the probability of success or reward and under such conditions decisions are made on the basis of action values, calculated from the expected probability that a candidate action will lead to reward multiplied by the reward value [9] , [10] , [11] . Choosing between actions requires, therefore, the ability to compare action values, a comparison that should occur, logically, as a precursor to choice, serving as an input into the decision-making process. Nevertheless, despite the importance of this process, it is not known how such comparisons are made, and where in the brain these comparisons are implemented to guide action selection [12] . Conventionally, action values have been compared based on a difference score between the two values (for example, Q Left − Q Right in reinforcement-learning models [10] , [11] ) [13] , [14] . Although computationally straightforward, this approach can be sub-optimal because it requires the accurate estimation of the value of all available actions before the comparison can be made [15] . Ultimately, what matters to the agent is not necessarily the absolute difference in action values but which action has the greater value. As such, to make a decision, it is often sufficient to calculate the likelihood of an action being better than alternatives, rather than calculating by how much. As an alternative to the difference score, therefore, actions could be compared based on their relative advantage; that is, the probability that one action’s value is greater than the alternate action [16] , that is, P ( Q Left > Q Right ). The relative advantage ( P ) is less informative than the difference because it provides no information regarding the amount by which Q Left is greater than Q Right ; however, P is also more efficient because it is only necessary to calculate the relative advantage of taking an action without having to determine the value of the inferior action, and this is sufficient to optimally guide choice [3] , [17] . Studies to date have reported neural signals related to action value (that is, Q Right , Q Left ) in the caudate and efferent motor regions of the cortex [14] , [18] , [19] , [20] , [21] . However, few studies have reported neural signals related to the comparison of these values. Single-unit studies in monkeys have gone to some length to isolate action values from stimulus values using free-response tasks involving distinct motor actions instead of visual stimuli to discriminate options [18] , [20] . Using this approach, values related to the reward contingency of the separate actions have been distinguished in different striatal projection neurons. However, relatively few caudate neurons appear to represent the difference between action values [20] . Human neuroimaging studies have distinguished action values in motor regions of the cortex, such as the premotor cortex and supplementary eye field [13] , [14] , [21] ; however, only two studies have reported signals representing the difference between options and these studies involved choices between discriminative cues [13] , [14] . Consequently, it is unknown the extent to which these neural signals reflect differences in action values or learned stimulus values. Accordingly, we assessed the comparison of action values in an unsignalled choice situation, using a free-response test, to eliminate any potential influence of stimulus values on the comparison process. In each block, we programmed one response with a slightly higher reward contingency to produce realistic differences in action values, and participants had to learn which of the two actions was superior via feedback (note that because we manipulate reward contingency and not reward magnitude, contingency and value are effectively equivalent in our study). We distinguished two alternate computational signals comparing action values at each response: P representing the probability the left action was more likely to lead to reward than the right action ( Q Left > Q Right ); and D representing the difference between each action’s value ( Q Left − Q Right ). It is important to recognize that, although both models can potentially discriminate the best choice, we were concerned here to establish (i) whether P adds any advantage in predicting choice over D ; (ii) which model best predicts both choice performance and the changes in BOLD signal associated with those choices and (iii) whether any such region modulates choice-related activity in the motor cortex, representing the output of the decision process. The results show that actions are chosen on the basis of P values, that right dorsolateral prefrontal cortex (dlPFC) activity tracks these values and also modulates motor cortex activity in an action-specific manner. The relative advantage of an action appears, therefore, to be an important input into the decision-making process enabling action-selection. Behavioural choices and causal ratings track the best action Participants freely chose between two actions (left or right button presses) for a snack food reward (M&M chocolates or BBQ-flavoured crackers) in 40-s interval blocks ( Fig. 1a ). One action–outcome contingency (action value) was always higher than the other action; however, the identity of the high-value action varied across blocks so participants had to learn anew which action led to more rewards. The difference between action values also varied from large to small across blocks so the task difficulty ranged from easy (large) to difficult (small) conditions. We measured response rates on each action, as well as subjective causal ratings (0–10) for each action after each block. Across conditions, each participant selected the higher-value action more often than the low-value action ( Fig. 1b ; main effect of action contingency F =34.62, P <0.001). Causal judgments also closely reflected the differences in action value of each block ( Fig. 1c ; main effect of action contingency F =42.26, P <0.001. 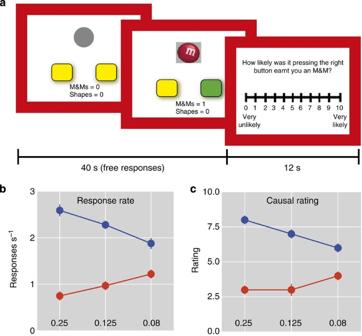Figure 1: Experimental stimuli, behavioural choices and causal ratings. (a) Before the choice, no stimuli indicated which button was more likely to lead to reward. When the participant made a choice, the button chosen was highlighted (green) and on rewarded trials the reward stimulus was presented for 1,000 ms duration. After each block of trials, the participant rated how causal each button was. (b) Mean response rate (responses per second) was higher for the high-contingency action (blue) over low-contingency action (red) in each condition. (c) Causal ratings were higher for the high-contingency action (blue) over low-contingency action (red) in each condition. Response rate and causal rating significantly varied with contingency,P<0.001. Vertical bars represent s.e.m. Figure 1: Experimental stimuli, behavioural choices and causal ratings. ( a ) Before the choice, no stimuli indicated which button was more likely to lead to reward. When the participant made a choice, the button chosen was highlighted (green) and on rewarded trials the reward stimulus was presented for 1,000 ms duration. After each block of trials, the participant rated how causal each button was. ( b ) Mean response rate (responses per second) was higher for the high-contingency action (blue) over low-contingency action (red) in each condition. ( c ) Causal ratings were higher for the high-contingency action (blue) over low-contingency action (red) in each condition. Response rate and causal rating significantly varied with contingency, P <0.001. Vertical bars represent s.e.m. Full size image The relative advantage and the Q difference guides choice We fit a Bayesian learning model, based on the relative advantage, to each subjects’ choice responses, which allowed us to generate P , that is, which action was more likely to result in reward. We also fit a Q-learning model to each individual subject using the maximum likelihood estimation method to generate D , that is, the difference between action–outcome contingencies ( Q Left and Q Right ). In addition, we generated a hybrid model in which choices are guided by both Q -learning and the relative advantage model (see Supplementary Fig. 1 for the negative log likelihoods). The results of a likelihood ratio test indicated that the hybrid model provided a better fit to participant choices than Q -learning, after taking into account the difference in number of parameters ( Table 1 ). This shows the relative advantage model accounted for unique variance in the subject choices over Q -learning alone. Individual model fit statistics and parameters are provided in Supplementary Table 1 . Table 1 Model comparisons between the hybrid model and its special cases. Full size table Inspection of the time course of P and D values across the session revealed they both discriminated the best action ( Fig. 2a ). However, the D signal quickly decayed towards the programmed difference in contingency in each block, which was usually small (that is, <0.2), whereas the relative advantage of the best action ( P ) was sustained across the block. To determine whether P was more predictive of choice when the difference in action values was small (that is, at intermediate values of D near or equal to zero), we compared the predictive value of P and D over choice at different levels of P and D in a logistic regression. 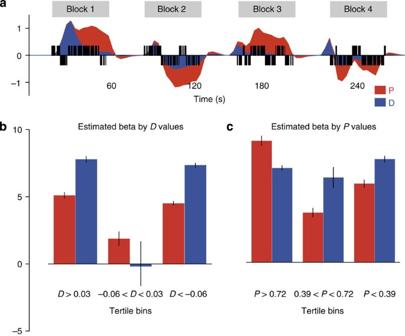Figure 2: Model valuesPandDpredict choices. (a) Trial-by-trial example of the actual choices made by Subject 7 (black vertical bars: left actions upward, right actions downwards), and the model-predicted values in arbitrary units forP(red) andD(blue) across the first four blocks (from easy to hard). NoticePrepresents a sustained advantage across each block, whileDdecays towards the experimental contingency in each block. (b) The regression weights ofP(red) andD(blue) values across tertile bins ofDvalues showing that as the difference inQLeftandQRightapproaches zero (middle tertile ofDvalues) onlyPvalues significantly predict choice. (c) Regression weights ofPandDacross tertile bins ofPvalues showing thatPandDare both significant predictors of choice across all tertiles ofP. Figure 2b shows we were able successfully to identify conditions under which P and D are differentiated: at small differences in action values (the middle tertile of D values), P was a significant predictor, whereas D was not. Conversely, Fig. 2c shows that P and D were significant predictors across all tertiles of P values (ps<0.001). This result confirms that when choices were made in the presence of small differences in action value, P values better discriminated the best action. Figure 2: Model values P and D predict choices. ( a ) Trial-by-trial example of the actual choices made by Subject 7 (black vertical bars: left actions upward, right actions downwards), and the model-predicted values in arbitrary units for P (red) and D (blue) across the first four blocks (from easy to hard). Notice P represents a sustained advantage across each block, while D decays towards the experimental contingency in each block. ( b ) The regression weights of P (red) and D (blue) values across tertile bins of D values showing that as the difference in Q Left and Q Right approaches zero (middle tertile of D values) only P values significantly predict choice. ( c ) Regression weights of P and D across tertile bins of P values showing that P and D are both significant predictors of choice across all tertiles of P . Full size image Dorsolateral prefrontal cortex tracks the relative advantage To identify the neural regions involved in the computation of the relative advantage values that guided choice, we defined a stick function for each response and parametrically modulated this by P in a response-by-response fashion for each participant. As we used a free-response task and the interval between choices was not systematically jittered, we cannot determine whether the model variables had separate effects at the time of each choice (or between choice and feedback). We can only determine whether neural activity was related to the time course of the model variables across the 40-s block as subjects tried to learn the best action (for example, Fig. 2a ). An SPM one-sample t -test with the parametric regressor representing P revealed neural activity positively related to P in a single large cluster in the right middle frontal gyrus, with the majority of voxels overlapping BA9 (dlPFC [22] , [23] ; peak voxel: 44, 25, 37; t =5.98, family-wise cluster (FWEc) P =0.012). Figure 2a shows the cortical regions where the BOLD response covaried with the P values of each response, implicating these regions in encoding the relative likelihood that the left action is best ( Q Left > Q Right ). 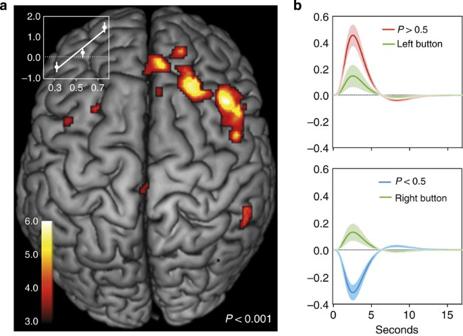Figure 3: Right dlPFC tracked the relative advantage signal. (a) Cortical regions correlated with the relative advantage signal (P). Only the right dlPFC (BA9) was significant FWEcP<.05. Inset, per cent signal change in the right dlPFC was linearly related toP. (b) Fitted responses in arbitrary units showing action-specific modulation of brain activity (red and blue) byP, as well as non-specific activity due to left and right actions (button presses) in the right dlPFC. Figure 3a inset shows that the per cent signal change at the peak voxel in the right dlPFC cluster was linearly related to the magnitude and direction of P , after splitting the P values into three separate and equal-sized bins (high, medium and low tertiles) and calculating the mean local per cent signal change in each bin using rfxplot [24] . Figure 3b shows the right dlPFC distinguished when the relative advantage of the left action was greater than the right ( P >0.5) and when the right action was greater than the left ( P <0.5), alongside the BOLD response when the left and right button press occurred. Comparison of the fitted response with the high and low P values relative to button presses clearly showed that the right dlPFC activity did not simply reflect the motor response (button press), because the direction of the BOLD signal discriminated between high and low P values, but not action choices. Figure 3: Right dlPFC tracked the relative advantage signal. ( a ) Cortical regions correlated with the relative advantage signal ( P ). Only the right dlPFC (BA9) was significant FWEc P <.05. Inset, per cent signal change in the right dlPFC was linearly related to P . ( b ) Fitted responses in arbitrary units showing action-specific modulation of brain activity (red and blue) by P , as well as non-specific activity due to left and right actions (button presses) in the right dlPFC. Full size image Differentiating action contingencies and action policies We tested for regions representing the difference between action values ( D ) in a similar but separate GLM. As P and D were highly correlated for some subjects (for example, Pearson r =0.86 for Subject 01; see Supplementary Table 2 for a complete list), a separate GLM was used to avoid the orthogonal transformation of parametric modulators in SPM and preserve the integrity of the signal. In the same manner as described above for P values, we defined a stick function for each response and parametrically modulated this by D in a response-by-response fashion for each participant. An SPM one-sample t -test of this modulator revealed that no clusters met our conservative correction for multiple comparisons (FWEc<0.05). The peak voxel occurred in a marginally non-significant cluster in the right inferior parietal lobe (BA40: 38, -38, 34; t =5.58, FWEc=0.066). The effect of the D signal in the right dlPFC at the same coordinates identified for P (44, 25, 37) was t =2.99, FWEc=0.236. The failure to find an action-specific delta signal in the brain is consistent with at least one other study that also reported no spatially coherent effect of delta signal [13] . The Q -learning model also contains a policy function that maps value differences ( D ) to choice, π . Policy ( π ) represents the probability of taking each action on the basis of the size of the difference between actions, and so it may characterize an alternative to the relative advantage signal. For this reason we also tested for brain activity correlating with π in a separate GLM. An SPM one-sample t -test of this modulator revealed that no clusters exceeded our cluster-level correction (FWEc=0.37). The absence of a D or policy signal in prefrontal regions does not support the results of our behavioural modelling, which suggested that under large contingency differences (that is, large D values) subject’s choices were predicted by D . Our behavioural modelling also showed that large D values were rare in our task, so there may not have been sufficient power to detect fMRI-related changes in the current test. To formally determine which of the variables ( P , D or π ) provided the best account of neural activity in the right dlPFC, we performed a Bayesian model selection analysis [25] , [26] . Specifically we used the first-level Bayesian estimation procedure in SPM8 to compute the log evidence for both signals in every subject in a 5-mm sphere centred on the right dlPFC (44, 25, 37). Subsequently, to model inference at the group level, we applied a random effects approach to construct the exceedance posterior probability (that is, how likely a specific model generated the data of a random subject) for each signal in the right dlPFC. The results found the P signal provided a better account of neural activity in the right dlPFC than the D or π signal (exceedance posterior probabilities 0.84, 0.12, 0.04, respectively). Thus, the weight of evidence suggests that right dlPFC activity represents the likelihood of the best action, rather than the difference in action–outcome contingencies or a policy based on that difference. Chosen action values and the ventromedial prefrontal cortex We also tested whether the contingency of the chosen action could be distinguished in separate brain regions ( Q Chosen ). This test represents an important (positive) control since chosen action values, or expected reward values, have been widely reported in the ventromedial prefrontal cortex. However, chosen values are not the focus of the present study as they can only be established post-decision and so cannot serve as an input into the decision process. The peak voxel corresponding to the chosen value in the whole-brain occurred in a single cluster in the medial frontal gyrus in the orbitofrontal cortex (OFC: −11, 47, −11; t =23.73, FWEc P <0.0001). 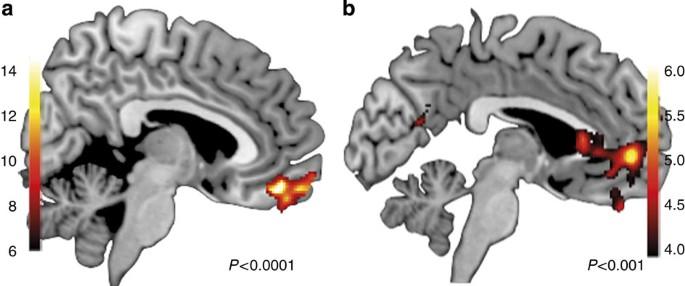Figure 4: Ventromedial PFC tracked post-choice values. (a) Peak voxel in the medial orbitofrontal cortex region correlated with the chosen action value (expected reward). (b) Peak voxel in the ventromedial prefrontal cortex correlated with the unchosen action value. Figure 4a shows the extent of the cluster extending rostrally to the ventromedial prefrontal cortex. No other regions were significant (FWEc P >0.05). To further explore the effect of post-decision values, we tested the contingency of the unchosen action. Figure 4b shows a cluster slightly dorsal to the effect of chosen action in the anterior cingulate (AC: 3, 50, −2; t =5.76, FWEc P =0.001). The fact that chosen action values occurred in a cortical area regionally distinct from the action-value comparisons we found in the right dlPFC indicates we were able to successfully distinguish pre-choice and post-choice values. The finding of chosen action values in the ventromedial prefrontal cortex replicates a number of other findings [12] , [14] , [19] , [27] , [28] , [29] , [30] , [31] , [32] , [33] , and is consistent with the suggestion that the output of the decision process is passed to ventral cortical regions for the purpose of updating action values, perhaps via reinforcement learning. Figure 4: Ventromedial PFC tracked post-choice values. ( a ) Peak voxel in the medial orbitofrontal cortex region correlated with the chosen action value (expected reward). ( b ) Peak voxel in the ventromedial prefrontal cortex correlated with the unchosen action value. Full size image Action control of motor cortex is modulated by right dlPFC To compare the role of the regions indicated by the GLM analyses of action-value comparisons (right dlPFC) and chosen values (OFC) on the control of actions in the motor cortex, we compared competing dynamic causal models using DCM10 (ref. 34 ) and tested inferences on model space using Bayesian model selection. The goal was to determine whether motor cortex activity, representing the output of the decision process, was better explained by action-specific modulation from the right dlPFC or the OFC. We extracted activation time courses from each individual’s peak voxel in the right dlPFC, OFC and motor cortex, and constructed eight different models of potential connectivity between each area ( Supplementary Fig. 2 ), as well as a null model with no modulation (model 0). Each model varied the location of action-specific modulation of motor cortex activity, as well as the driving inputs to the dlPFC and OFC. The results of the Bayesian model selection ( Fig. 5 ) established that the winning model was model 1 ( Fig. 5a inset), with an exceedance probability of 99.02 per cent ( Fig. 5a ). Only this model specified action-specific modulation of the motor cortex from the right dlPFC in combination with P values as the driving input. The expected probability, that is, how likely a specific model generated the data of a random subject, for each model is shown in Fig. 5b . The expected probability for the winning model (model 1) was 54.15 per cent, meaning that evidence for model 1 is likely to be obtained in the majority of any randomly selected subjects, and indicates the generalizability of these findings. Overall, the results of the DCM analysis provided clear evidence that the action executed by the motor cortex is guided by the action-value comparisons computed by the right dlPFC likely via the caudate. Indeed, ROI analysis of caudate activity in the current study confirmed that, as described previously, the anterior caudate covaried with the experienced correlation between response rate and reward [32] (peak voxel in ROI: 16,18,4; t =6.74, P =0.002 svc—see Supplementary Fig. 3 ). 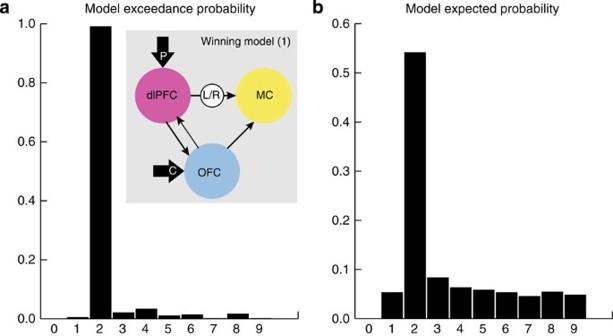Figure 5: Right dLPFC modulated motor cortex. (a) Probability that one model is more likely than any other model. Inset, winning model with dlPFC modulating motor cortex activity in an action-specific manner (b) How likely a specific model generated the data of a random subject. Figure 5: Right dLPFC modulated motor cortex. ( a ) Probability that one model is more likely than any other model. Inset, winning model with dlPFC modulating motor cortex activity in an action-specific manner ( b ) How likely a specific model generated the data of a random subject. Full size image A critical question in decision neuroscience is how and where in the brain actions are compared to guide choice [12] . The present results provide evidence that actions are compared on the basis of their relative advantage ( P ) in a two-armed bandit task, that is, the probability that an action is more likely to lead to reward than another action, and this comparison is utilized by the right dlPFC to control choice behaviour. Activity in the right dlPFC tracked the relative advantage ( P ) over other comparison signals (for example, the relative strength of the best action, D ), which also could be used to predict choice. Furthermore, activity in this region was not differentially modulated by post-choice values, such as the chosen action contingency, or the actions taken (for example, a right or left button press). Effective connectivity analysis showed the right dlPFC-modulated activity in the motor cortex, the major output pathway for choice behaviour, in an action-specific manner. As a consequence, this directional signal may represent an important input into the decision-making process, enabling the subject to choose the course of action more likely to lead to reward. The dlPFC is also connected with the orbitofrontal cortex, which represents important value signals such as the expected reward value [29] . In particular, we found that activity in the OFC tracked the chosen action contingency, which is equivalent to the expected reward value in this task. A number of studies have found expected reward signals in this region [14] , [27] , [28] , [29] , [30] , [31] , [32] , [33] , as well as the medial prefrontal cortex [32] , [35] and amygdala [36] . Some studies have also found that the reward signal in the OFC precedes the dlPFC response [37] , which implies that reward value information is relayed from the OFC to the dlPFC. Our DCM analysis did not indicate this direction of effect (albeit, the parameters of our task did not provide sufficient temporal resolution to distinguish the order of effect). However, expected reward values are necessary to compute a prediction error in model-free reinforcement learning to update action values before the next trial [10] . As such, they are quite distinct from action values and cannot serve as inputs to the comparison process because they reflect the value of actions already selected in the decision, that is, expected reward values reflect decision output rather than input, which was the focus of the present study. We also tested the relative roles of the right dlPFC and the OFC in action selection by comparing DCMs with relevant variations in action-specific modulation between regions. The most likely models, given our data, indicated the dlPFC modulated motor cortex activity in an action-specific manner. We failed to find any substantive evidence for models in which the right dlPFC modulated OFC activity, or the OFC modulated motor cortex activity. It is worth noting that effective connectivity does not reflect or require direct connections between regions, as the effective connectivity can be mediated polysynaptically [38] . We speculate the effect of the right dlPFC on motor cortex is mediated via connections with the caudate, given the evidence of anatomical connections between these regions [39] , [40] , and the caudate’s established role in goal-directed choice [41] . We did not, however, observe action-specific value signals in the dorsal striatum, as has been reported in single-unit studies in primates [18] , [20] , [42] . Nevertheless, it is likely that connections between the dlPFC, the OFC and the striatum [32] , [35] participate in a circuit to compare action values, select actions and update action values once a choice has been made. Single-unit studies in primates have found that a number of neurons in the dlPFC are predictive of an animal’s decision in choices between discriminative cues [37] , [43] , [44] , and stimulation of dlPFC neurons can bias a decision [45] , [46] . A prevalent idea about the functional specialization of the prefrontal cortex is that the OFC processes information about reward value [31] , [47] , [48] , whereas the dlPFC functions in the selection of goals and actions [44] , [49] , [50] . The dlPFC is heavily interconnected with areas responsible for motor control [51] , [52] , [53] and so may represent an area where information about reward value and action converges to allow action comparisons to take place; however, there are other regions that could integrate reward information and motor action, such as anterior cingulate [54] and the parietal cortex [5] . Overall, our results extend the established role of the dlPFC in the selection of goals and actions to include the computational comparison of action values. Furthermore, the dlPFC determines that this comparison occurs in terms of relative likelihood of the best action rather than the relative strength of the best action. Evidence that action-value comparisons occur in the human brain has been scarce [12] . Wunderlich et al . [21] identified action-specific values in the supplementary motor cortex and premotor area using very distinct motor actions in order to discriminate between choices (for example, hand versus eye movements). Wunderlich et al . [21] also found that post-choice values (unchosen over chosen values) were compared in the anterior cingulate cortex, where we found unchosen action values were tracked. Although such results clearly distinguish separate action-specific value signals in different regions of the motor cortex, the regressors tested involved post-choice values and so were not precursors to choice. Evidence of a neural signal representing the difference between Q values and that could act as an input into a decision comparator has been provided by another study using magnetoencephalography [14] . This study reported that the direction of comparison was contralateral to the hemisphere of the delta signal (that is, Q Contralateral − Q Ipsilateral ); however, whether this comparison reflected action values or stimulus values is uncertain due to the discriminative cues provided by the task. Even so, it is worth noting that the comparison we found (that is, Q Left > Q Right ) in the right prefrontal cortex is consistent with evidence that decision values occur in the contralateral hemisphere [14] , [19] . We did not find the inverse direction in the left hemisphere (that is, Q Right > Q Left ), presumably because our participants only used their right hand to respond; however, there are many differences in the task and temporal dynamics of the image data that may account for this. Ultimately, a single bidirectional signal is sufficient to guide choice, so the unilateral effect we found may reflect an innate bias in right-handed actions or right-handed subjects seeking neural efficiency. Our modelling of choice performance implied people used more than one strategy for selecting between actions—both P and D were predictive of choice; however, when the difference between action values ( D ) was small, participants used the relative advantage ( P ) to select the best action ( Fig. 2b ). We cannot determine from our data alone whether the use of relative advantage ( P ) occurs generally or only when D is difficult to compute or uncertain. Likewise, we cannot determine whether the right dlPFC computes the best action on the basis of each response or whether P is computed over a set of responses. However, as discussed by others (and above) [3] , [55] , [56] , when action outcomes are uncertain, a good heuristic solution in a multi-armed bandit problem is to restrict estimation of each action contingency until the values indicate a likely winner rather than to continue estimating each action contingency after an advantage is known. This strategy is represented by the relative advantage comparison, which has also been shown to scale well when the number of choices increases above two (for example, 10-arm bandit [3] ). Thus, the fact that the neural signal in the dlPFC reflected P , even under conditions in which D was predictive ( Fig. 2c ), represents a dissociation consistent with a unique role for this neural region in this task. To our knowledge, this is the first demonstration of such a computational comparison in humans or other animals. Finally, our results have implications for neural models of decision-making. We used a model-based form of Bayesian learning that directly estimates the action contingencies (state transition probabilities) from the conditional probabilities of reward, rather than a model-free approach that uses prediction errors to estimate action values. The model-based method was chosen on the basis of prior evidence that the cortical regions of interest are sensitive to contingency changes [32] , [35] . Although our modelling was not able to determine conclusively whether or not people adopted a model-free or model-based strategy, the subjective causal ratings of each action corresponded closely with the action contingencies, demonstrating participants were aware of the contingencies in each block. Under such conditions, people may be more likely to adopt a model-based strategy, rather than an implicit model-free strategy. Recent model-based accounts of decision-making assume uncertainty around each action/stimulus value determines how quickly the value is updated (that is, the learning rate) [57] , [58] . In such models, uncertainty is represented separately in the decision process, as well as the brain [58] , [59] . By contrast, the relative advantage signal we found summarizes the difference between action values as well as the uncertainty around them in a single value. The implication for models of decision-making is that action values and uncertainty are not always represented separately at the decision-point, but instead are combined to indicate the best action. In conclusion, the present report provides direct evidence of an action-specific comparison signal in the human cortex. It is striking that existing studies of action-specific values using human fMRI have not previously succeeded in revealing a comparison signal in the cortex that is regionally homogenous. As such, these results may also suggest that the comparison process revealed here is a unique feature of goal-directed decision-making and may not reflect a more general action-value comparison strategy based, for example, on predictive stimuli. Subjects Twenty-three right-handed subjects (11 females), age range 17–32 years, were recruited for the study. Three participants were removed due to excessive head movement (> 2 mm). Thus, n =20, and all participants were unmedicated, free of neurological or psychiatric disease and consented to participate. The study was approved by the Human Research Ethics Committee at Sydney University (HREC no. 12812). After scanning, all participants were reimbursed $45 in shopping vouchers, in addition to the snack foods that they earned during the test session. Stimuli and task The instrumental learning task ( Fig. 1a ) involved choosing between two action, left and right button presses, for a snack food reward (M&M or BBQ shape) and was conducted in a single replication. Participants were instructed to press the left or right button with their right hand, and try to earn as many snacks as they can. Actions were taken by pressing separate buttons on a Lumina MRI-compatible two-button response pad. The session was arranged in 12 blocks of 40-s duration, and in each block the participant responded freely for reward [32] , [35] . Reward was indicated by the presentation of a visual stimulus depicting the outcome (for example, M&M) for 1,000 ms and the visual tally of the total number of rewards was increased. No feedback was provided in the absence of a win. At the end of each block, participants were given 12 s to rate how causal each action was with respect to the outcome on a visual analogue scale from 1 to 10. Blocks differed according to their outcome contingencies on the left and right actions but only one outcome was available in each block. Thus, there were six pairs of action contingencies [0.25, 0.05], [0.05, 0.25], [0.05, 0.125], [0.125, 0.05], [0.08, 0.05] and [0.05, 0.08], and each was repeated twice, once for each outcome (M&M and BBQ shapes). Importantly, no cue indicated which action was the high contingency action at the time of the decision. As the contingencies changed between blocks and the beginning of each block was cued, participants had to learn anew within each block which action led to more rewards. At the end of the session, participants received the total number of snack foods they had earned. Bayesian learning model To estimate the action contingencies on the basis of experience for each participant, we used a Bayesian learning method. This method treats the contingency as a random variable, and calculates its probability distribution. We assumed the probability of receiving reward by executing each action is a binomial distribution with parameters p Left and p Right for left and right actions, respectively. These probabilities were then represented with Beta distributions: We assumed uninformative priors over the parameters that roll off at boundaries, (α 1 , α 2 , β 1 , β 2 =1.1). After executing each action i ( i= Left, Right) and receiving the outcome, the underlying distributions update according to Bayes rule: Where r =1 is reward, and r =0 is non-reward. Finally, we define delta as Δ= p Left − p Right . By denoting: We will have: Where Where μ and σ 2 are mean and variance of Δ′, respectively, and can be calculated in a straightforward manner. Based on this, the relative advantage is equivalent to: Hereafter, we will represent the relative advantage P (Δ>0) as P . In this manner, we modelled the action-specific comparisons that allow the decision-maker to make choices without perfect knowledge of the contingencies. In fact, the relative advantage will change as the certainty around each contingency estimate changes, as well as the distance between the most likely estimates of each contingency changes. The relative advantage also reflects the assumption that once an action is estimated to be more likely to lead to reward than the other action with absolute certainty, that is, P =1, the advantage does not further increase with increases in contingency. Q-learning model As an alternative to the Bayesian learning model, we used a Q-learning method, which estimates a value for each action. After executing each action i ( i =left, right) and receiving outcome, the value of each action updates according to the temporal-difference rule: where α is the learning rate. If the action is rewarded r =1, otherwise r =0. We defined the difference between action values as follows: The values for Q Left and Q Right were initially set to zero. Action selection To model individual choices according to experience, we assumed that the probability of taking each action is proportional to its values, and its relative advantage over the other action. Using the softmax rule, the probability of taking the left action, π(left) will be: where τ p and τ q are the ‘inverse temperature’ parameters, and controls exploration–exploration balance. τ p and τ q control the contribution of the P and Q values to the choice probabilities, respectively. k ( A ) is the action preservation parameter and captures the general tendency of taking the same action as the previous trial [60] , [61] . k ( A ) is equal to k when the chosen action in the previous trial is the same as A , and otherwise it is equal to zero. We generated the model described in equation (1) as well as two nested models by setting τ p=0 and τ q=0 , and fitting them to the subject’s behaviour individually, using the maximum-likelihood estimate. For optimization we used the Ipopt software package [62] . We compared models using the likelihood ratio test and measured the overall goodness of fit by computing pseudo R 2 using the best fit model for each subject. Pseudo R 2 was defined as ( R – L )/ R for each subject, where L and R are the negative log likelihoods of the hybrid model (1) and a null model of random choices, respectively [28] . For the purpose of generating model-predicted time series for fMRI regression analysis, D and π values for each individual were generated using the restricted model τ p =0 with parameters ( τ q , α and k ) set to the maximum-likelihood estimate over the whole group [63] , similar to other work in this field [64] . Simulations determined these Q-learning parameters could be accurately recovered from choice data ( Supplementary Table 3 ). We also tested D values using the hybrid model but since it made no difference to the final result, only the test of the nested model values are provided here. P values were generated using the restricted model τ q=0 and are independent of model parameters (note: P values generated from the hybrid model and nested model did not differ). Each individual’s P and D values were entered as a parametric modulator of responses in the fMRI analysis below to identify brain areas where the value comparison computation might be carried out. fMRI data acquisition Gradient-echo T2*-weighted echo-planar images (EPI) were acquired on a Discovery MR750 3.0T (GE Healthcare, UK) with a resolution of 1.88 × 1.88 × 2.0 mm. Fifty-two slices were acquired (echo time 20 ms; repetition time 3.0 s; 0.2 mm gap) in an interleaved acquisition order. The acceleration factor (ASSET) was 2, which allowed data acquisition from a whole-brain volume with 240 mm field of view angled 15° from AC-PC in each subject to reduce signal loss. In each session 260 images were collected (~13 min each). Image analysis Preprocessing and statistical analysis were performed using SPM8 (Wellcome Trust Centre for Neuroimaging, London, UK; www.fil.ion.ucl.ac.uk/spm ). The first four images were automatically discarded to allow for T1 equilibrium effects, then images were slice-time-corrected to the middle slice and realigned with the first volume. The mean whole-brain image was then normalized to MNI space and the resulting normalization parameters applied to the remaining images. Images were then smoothed with a Gaussian kernel of 8-mm FWHM. Based on our behavioural analysis, we estimated several general linear models (GLM) for each individual. Block duration, rating periods, responses and rewards were included as separate subject-specific regressors in each GLM. Responses were parametrically modulated by the relative advantage value P in the first GLM. Separate GLMs modulated responses by D (the expected value of the difference between action contingencies), which replicates methods used in other reports [13] . We also tested the chosen action contingency as this represents the expected reward value of the chosen action and serves as a useful comparison to other reports of expected values in the prefrontal cortex [30] , [65] . The chosen action contingency was calculated as the experienced contingency between the current action and its accumulated rewards since the beginning of the block. The resulting stimulus functions were convolved with the canonical hemodynamic response function. Regression was performed using standard maximum likelihood in SPM. Low-frequency fluctuations were removed using a high-pass filter (cutoff 128 s) and remaining temporal autocorrelations were modelled with a two-parameter auto-regression model. To enable inference at the group level, we calculated second-level group contrasts using a one-sample t -test in SPM. Regions exceeding a voxel-wise threshold P <0.001, along with an FWEc threshold P <0.05 to correct for multiple comparisons are reported. As P and D are action-specific values, that is, a comparison of one action over another action, the values must provide a direction of comparison in order to ultimately guide action selection (for example, Q Left > Q Right or Q Right < Q Left ). Determining the direction of comparison each subject employed a priori was not possible, so we assumed a single direction of comparison for all subjects in a unidirectional t -test (SPM default) and then determined the direction of comparison by examining the eigenvariate of each subject at the group peak voxel. The neural responses from only three subjects had an inverse relationship with P and D relative to the rest of the group and reversing their direction did not change the imaging results, so we report here the results of our initial analysis, assuming the same direction for all subjects. Dynamic causal modelling To compare the role of the regions associated with action comparisons and choice on the control of choice behaviour in the motor cortex, we specified seven competing models of functional architecture using DCM10 (ref. 34 ) and tested inferences on model space using Bayesian model selection. The goal was to determine whether motor cortex activity, representing the output of the decision process, was better explained by action-specific changes in effective connectivity from the right dlPFC or the OFC, since both these regions were indicated in the GLM analysis of action comparisons and chosen action contingencies described above. The analysis was carried out in several steps [66] . First, activation time courses were extracted from each individual’s peak voxel within 5 mm of the global peak voxel coordinates of the group in each of three analyses: action-specific comparisons using the relative advantage values, peak MNI coordinates [+44, 25, 37]; the chosen action contingency, peak MNI coordinates [−11, 47, −11] and button presses (responses), peak MNI coordinates [−4, 25, 70]. Second, we specified eight different models of potential connectivity between each area, with varying locations of action-specific modulation of motor cortex activity ( Supplementary Fig. 2 , models 1–8), as well as a null model with no modulation (model 0). For each model tested, two driving inputs were included: (1) an input representing the relative advantage values to the right dlPFC and (2) an input representing the chosen action contingency to the OFC. As we wished to explain activity in the motor cortex in terms of connectivity, no driving input was included for the motor cortex. In addition, action-specific changes in coupling strength were modelled by specifying left and right button presses separately. Note, only models 1 and 2 ( Supplementary Fig. 2 ) included action-specific coupling between the right dlPFC and motor cortex. We then identified the best model using Bayesian model selection [67] . Briefly, this technique treats the models as random variables and computes a probability distribution for all models under consideration. This procedure permits the computation of the exceedance probabilities for each model, which represents the probability that each model is the most likely one to be correct. The exceedance probabilities add to one over the comparison set, and thus generally decrease as the number of models considered increases. How to cite this article: Morris R. W. et al . Action-value comparisons in the dorsolateral prefrontal cortex control choice between goal-directed actions. Nat. Commun. 5:4390 doi: 10.1038/ncomms5390 (2014).